Quantum criticality in electron-doped BaFe2−xNixAs2 A quantum critical point is a point in a system’s phase diagram at which an order is completely suppressed at absolute zero temperature ( T ). The presence of a quantum critical point manifests itself in the finite- T physical properties, and often gives rise to new states of matter. Superconductivity in the cuprates and in heavy fermion materials is believed by many to be mediated by fluctuations associated with a quantum critical point. In the recently discovered iron–pnictide superconductors, we report transport and NMR measurements on BaFe 2− x Ni x As 2 (0≤ x ≤0.17). We find two critical points at x c1 =0.10 and x c2 =0.14. The electrical resistivity follows ρ = ρ 0 + AT n , with n =1 around x c1 and another minimal n =1.1 at x c2 . By NMR measurements, we identity x c1 to be a magnetic quantum critical point and suggest that x c2 is a new type of quantum critical point associated with a nematic structural phase transition. Our results suggest that the superconductivity in carrier-doped pnictides is closely linked to the quantum criticality. In cuprate high temperature superconductors [1] and heavy fermion [2] compounds, the superconductivity is accompanied by the normal-state properties deviated from a Landau–Fermi liquid. Such deviation has been ascribed to the quantum critical fluctuations associated with a quantum critical point (QCP) [3] , [4] , whose relationship to the occurrence of superconductivity has been one of the central issues in condensed-matter physics in the last decades. In iron–pnictide high-temperature superconductors [5] , [6] , searching for magnetic fluctuations has also become an important subject [7] . Quantum critical fluctuations of order parameters take place not only in spatial domain, but also in imaginary time domain [8] , [9] . The correlation time τ 0 and correlation length ξ are scaled to each other, through a dynamical exponent z , τ 0 ξ z . Several physical quantities, such as the electrical resistivity and spin-lattice relaxation rate (1/ T 1 ), can be used to probe the quantum critical phenomena. For the quasiparticles scattering dominated by the quantum critical fluctuations, the resistivity scales as ρ T n . For a two-dimensional (2D) antiferromagnetic spin-density wave (SDW) QCP, the exponent n =1 is often observed [1] , [2] , [10] . On the other hand, for a 2D order with q =(0,0) where z =3, n =4/3 at the QCP [11] , [12] . Around a QCP, 1/ T 1 also shows a characteristic T -scaling [11] . BaFe 2− x Ni x As 2 is an electron-doped system [13] where every Ni donates two electrons in contrast to Co doping that contributes only one electron [14] . Therefore, Ni doping suffers less from disorder which is usually harmful for a QCP to exist. In this work, we find two critical points at x c1 =0.10 and x c2 =0.14, respectively. By NMR measurements, we identify x c1 to be a magnetic QCP and suggest that x c2 is a QCP associated with the tetragonal-to-orthorhombic structural phase transition. The highest T c is found around x c1 , which suggests that the superconductivity in the carrier-doped BaFe 2 As 2 is more closely tied to the magnetic QCP, while the unusual quantum criticality associated with the structural transition deserves further investigation. 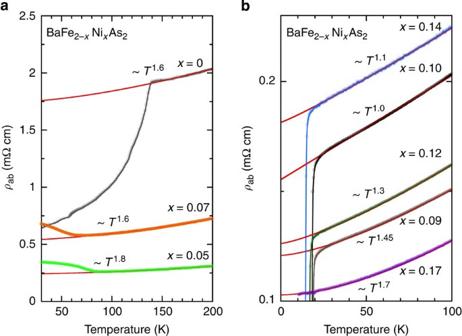Figure 1: The in-plane electrical resistivity. The in-plane electrical resistivityρabfor BaFe2−xNixAs2. The data in the normal state are fitted by the equationρab=ρ0+ATn(red curve). Electrical resistivity measurements Figure 1 shows the in-plane electrical resistivity data in BaFe 2− x Ni x As 2 for various x , which are fitted by the equation ρ ab = ρ 0 + AT n (for data over the whole temperature range, see Supplementary Fig. S1 and Supplementary Note 1 ). For a conventional metal described by the Fermi liquid theory, the exponent n =2 is expected. However, we find n <1.5 for 0.09≤ x ≤0.14. This is a notable feature of non-Fermi liquid behaviour. Most remarkably, a T -linear behaviour ( n =1) is observed for x c1 =0.10 and persists up to T =100 K. Another minimal n =1.1 is found for x c2 =0.14, which is in good agreement with a previous transport measurement [15] . An equally interesting feature is that both the residual resistivity ρ 0 and the coefficient A show a maximum at x c1 and x c2 as seen in Fig. 2a . The evolution of the exponent n with Ni content is shown in Fig. 2b . Figure 1: The in-plane electrical resistivity. The in-plane electrical resistivity ρ ab for BaFe 2− x Ni x As 2 . The data in the normal state are fitted by the equation ρ ab = ρ 0 + AT n (red curve). 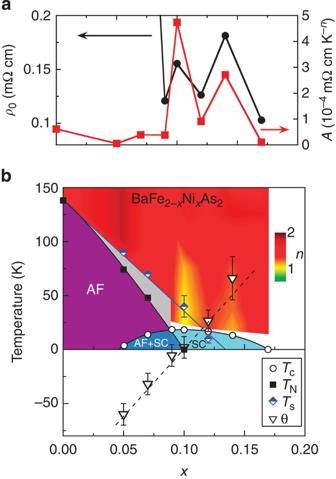Figure 2: The obtained phase diagram of BaFe2−xNixAs2. (a) The residual resistivityρ0and the coefficientAas a function of Ni-dopingx. (b) The obtained phase diagram of BaFe2−xNixAs2. TheTNandθare obtained from NMR spectra and 1/T1T, respectively. AF and SC denote the antiferromagnetically ordered and the superconducting states, respectively. The solid and dashed lines are the guides to the eyes. Colours in the normal state represent the evolution of the exponentnin the resistivity fitted byρab=ρ0+ATn. The light yellow region atx=0.10 shows that the resistivity isT-linear. The error bar forθis the s.d. in the fitting of 1/T1T. The error bar forTsrepresents the temperature interval in measuring the NMR spectra. Full size image Figure 2: The obtained phase diagram of BaFe 2− x Ni x As 2 . ( a ) The residual resistivity ρ 0 and the coefficient A as a function of Ni-doping x . ( b ) The obtained phase diagram of BaFe 2− x Ni x As 2 . The T N and θ are obtained from NMR spectra and 1/ T 1 T , respectively. AF and SC denote the antiferromagnetically ordered and the superconducting states, respectively. The solid and dashed lines are the guides to the eyes. Colours in the normal state represent the evolution of the exponent n in the resistivity fitted by ρ ab = ρ 0 + AT n . The light yellow region at x =0.10 shows that the resistivity is T -linear. The error bar for θ is the s.d. in the fitting of 1/ T 1 T . The error bar for T s represents the temperature interval in measuring the NMR spectra. Full size image NMR measurements We use NMR to investigate the nature of x c1 and x c2 . We identify x c1 to be a SDW QCP and suggest that x c2 is a tetragonal-to-orthorhombic structural phase transition QCP. 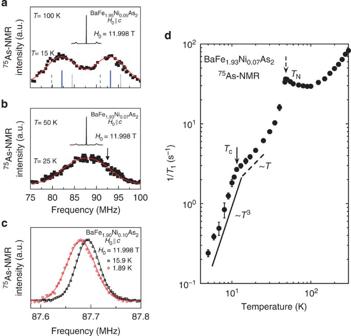Figure 3: NMR spectra with doping and temperature dependence of 1/T1at optimal doping. 75As-NMR spectra obtained by sweeping the frequency at a fixed external fieldH0=11.998 T applied along thecaxis. (a) The spectra above and belowTN=74 K forx=0.05. Solid, dashed and dotted lines indicate, respectively, the position of the central transition, left- and right-satellites, when an internal magnetic field develops. (b) The spectra above and belowTN=48 K forx=0.07. The red curve represents the simulations by assuming a Gaussian distribution of the internal magnetic field. The black arrow indicates the position at whichT1is measured belowTN. (c) The central transition line at and belowTcforx=0.10. The spectrum shift atT=1.89 K is due to a reduction of the Knight shift in the superconducting state. (d) The temperature dependence of 1/T1forx=0.07. The solid and dashed lines show theT3- andT-variation, respectively. The solid and dashed arrows indicateTcandTN, respectively. The error bar in 1/T1is the s.d. in fitting the nuclear magnetization recovery curve. Figure 3a,b display the frequency-swept spectra of 75 As NMR for x =0.05 and 0.07, respectively. The very narrow central transition peak above the antiferromagnetic transition temperature T N testifies a good quality of the samples. When a magnetic order sets in, the spectra will split into two pairs as labelled in Fig. 3a , due to the development of an internal magnetic field H int . For x =0.05, we observed two split broad peaks below T N =74 K. This is due to a distribution of H int , which results in a broadening of each pair of the peaks. Upon further doping, H int is reduced and its distribution becomes larger, so that only one broad peak can be seen below T N =48 K for x =0.07. Similar broadening of the spectra was also observed previously in a very lightly-doped sample BaFe 1.934 Ni 0.066 As 2 (ref. 16 ). For both x , the spectra can be reproduced by assuming a Gaussian distribution of H int as shown by the red curves. We obtain the averaged internal field H int =0.75 T at T =15 K for x =0.05, and H int =0.39 T at T =25 K for x =0.07. By using a hyperfine coupling constant of 1.88 T per μ B obtained in the undoped parent compound [17] , the averaged ordered magnetic moment S is deduced. As seen in Fig. 4 , the ordered magnetic moment develops continuously below T N , being consistent with the second-order nature of the phase transition. It saturates to 0.43 μ B for x =0.05, and 0.24 μ B for x =0.07, respectively. The ordered moment is smaller than that in the hole-doped Ba 1− x K x Fe 2 As 2 (ref. 18 ), which is probably due to the fact that Ni goes directly into the Fe site and is more effective in suppressing the magnetic order. Upon further doping, at x =0.09 and x =0.10, however, no antiferromagnetic transition was found, as demonstrated in Fig. 3c , which shows no splitting or broadening ascribable to a magnetic ordering. Figure 3: NMR spectra with doping and temperature dependence of 1/ T 1 at optimal doping. 75 As-NMR spectra obtained by sweeping the frequency at a fixed external field H 0 =11.998 T applied along the c axis. ( a ) The spectra above and below T N =74 K for x =0.05. Solid, dashed and dotted lines indicate, respectively, the position of the central transition, left- and right-satellites, when an internal magnetic field develops. ( b ) The spectra above and below T N =48 K for x =0.07. The red curve represents the simulations by assuming a Gaussian distribution of the internal magnetic field. The black arrow indicates the position at which T 1 is measured below T N . ( c ) The central transition line at and below T c for x =0.10. The spectrum shift at T =1.89 K is due to a reduction of the Knight shift in the superconducting state. ( d ) The temperature dependence of 1/ T 1 for x =0.07. The solid and dashed lines show the T 3 - and T -variation, respectively. The solid and dashed arrows indicate T c and T N , respectively. The error bar in 1/ T 1 is the s.d. in fitting the nuclear magnetization recovery curve. 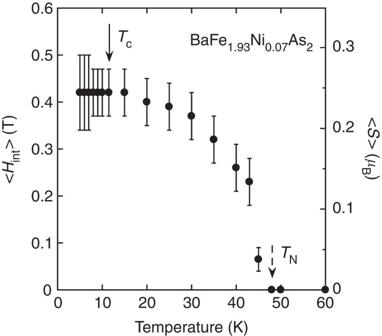Figure 4: The temperature dependence of the internal magnetic field and the ordered moment forx=0.07. Temperature dependence of the averaged internal magnetic fieldHint(left vertical axis) and the averaged ordered momentS(right vertical axis) forx=0.07. The solid and dashed arrows indicateTcandTN, respectively. The error bar represents the absolute maxima (minima) that can fit a spectrum. Full size image Figure 4: The temperature dependence of the internal magnetic field and the ordered moment for x =0.07. Temperature dependence of the averaged internal magnetic field H int (left vertical axis) and the averaged ordered moment S (right vertical axis) for x =0.07. The solid and dashed arrows indicate T c and T N , respectively. The error bar represents the absolute maxima (minima) that can fit a spectrum. Full size image The onset of the magnetic order in the underdoped regime is also clearly seen in the spin-lattice relaxation. Figure 3d shows 1/ T 1 for x =0.07, which was measured at the position indicated by the arrow in Fig. 3b , in order to avoid any influence from possible remnant paramagnetic phase, if any. As seen in Fig. 3d , a clear peak is found at T N =48 K due to a critical slowing down of the magnetic moments. Below T N , 1/ T 1 decreases down to T c . Most remarkably, 1/ T 1 shows a further rapid decrease below T c , exhibiting a T 3 behaviour down to T =5 K. Such a significant decrease of 1/ T 1 just below T c is due to the superconducting gap opening in the antiferromagnetically ordered state. This is clear and direct evidence for a microscopic coexistence of superconductivity and antiferromagnetism, as the nuclei being measured experience an internal magnetic field yet the relaxation rate is suppressed rapidly below T c . For x =0.10, as mentioned already, no antiferromagnetic transition was found. Namely T N =0. This is consistent with the extrapolation of the T N versus x relation that gives a critical point that coincides with x c1 =0.10, which is further supported by the spin dynamics as elaborated below. 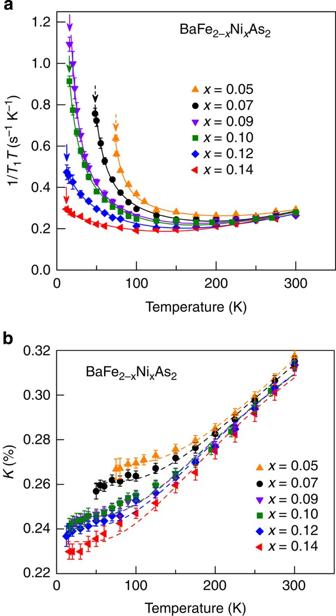Figure 5: The quantity 1/T1Tand the Knight shift. (a) Temperature dependence of 1/T1Tand (b) the Knight shiftKfor variousx. The solid line is a fitting of. The dashed curve is a fit toK=K0+Ks× exp(−Eg/kBT). The obtained parameters areEg/kB=620±40, 510±40, 370±30, 365±30, 350±30 and 330±30 K forx=0.05, 0.07, 0.09, 0.10, 0.12 and 0.14, respectively. The solid and dashed arrows indicateTcandTN, respectively. The error bar for 1/T1Tis the s.d. in fitting the nuclear magnetization recovery curve. The error bar forKwas estimated by assuming that the spectrum-peak uncertainty equals the point (frequency) interval in measuring the NMR spectra. Figure 5a shows the quantity 1/ T 1 T for 0.05≤ x ≤0.14. The 1/ T 1 T decreases with increasing T down to around 150 K, but starts to increase towards T N or T c . The increase at low T is due to the antiferromagnetic spin fluctuation , and the decrease at high T is due to an intraband effect . Namely, . A similar behaviour was also seen in Ba(Fe 1− x Co x ) 2 As 2 (ref. 19 ). We analyse the (1/ T 1 T ) AF part by the self-consistent renormalization theory for a 2D itinerant electron system near a QCP [11] , which predicts that 1/ T 1 T is proportional to the staggered magnetic susceptibility χ ″( Q ). As χ ″( Q ) follows a Curie–Weiss law [11] , one has . The intraband contribution is due to the density of state at the Fermi level, which is related to the spin Knight shift ( K s ) through the Korringa relation =constant [20] . The Knight shift was found to follow a T -dependence of K = K 0 + K s exp(− E g / k B T ) as seen in Fig. 5b , where K 0 is T -independent, while the second is due to the band that sinks below the Fermi level [21] , [22] . Correspondingly, we can write . The resulting θ is plotted in Fig. 2b . Note that θ is almost zero at x =0.10, which yields a constant 1/ T 1 above T c as seen in Fig. 6 . The result of θ =0 means that the staggered magnetic susceptibility diverges at T =0, indicating that x =0.10 is a magnetic QCP. Therefore, the exponent n =1 in the resistivity is due to the magnetic QCP (Generally speaking, scatterings due to the magnetic hot spots give a T -linear resistivity [11] , but those by other parts of the Fermi surface will not [23] , [24] . In real materials, however, there always exist some extent of impurity scatterings that can connect the magnetic hot spots and other parts of the Fermi surface as to restore the n =1 behaviour at a magnetic QCP). Figure 5: The quantity 1/ T 1 T and the Knight shift. ( a ) Temperature dependence of 1/ T 1 T and ( b ) the Knight shift K for various x . The solid line is a fitting of . The dashed curve is a fit to K = K 0 + K s × exp(− E g / k B T ). The obtained parameters are E g / k B =620±40, 510±40, 370±30, 365±30, 350±30 and 330±30 K for x =0.05, 0.07, 0.09, 0.10, 0.12 and 0.14, respectively. The solid and dashed arrows indicate T c and T N , respectively. The error bar for 1/ T 1 T is the s.d. in fitting the nuclear magnetization recovery curve. The error bar for K was estimated by assuming that the spectrum-peak uncertainty equals the point (frequency) interval in measuring the NMR spectra. 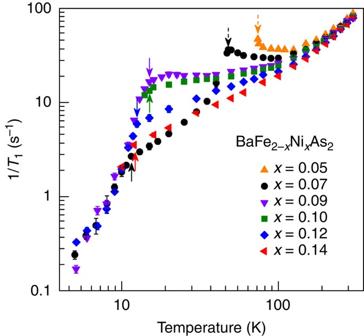Figure 6: The 1/T1for all the superconducting samples. The temperature dependence of the spin-lattice relaxation rate 1/T1for variousxof BaFe2−xNixAs2. The solid and dashed arrows indicateTcandTN, respectively. The error bar is the s.d. in fitting the nuclear magnetization recovery curve. Full size image Figure 6: The 1/ T 1 for all the superconducting samples. The temperature dependence of the spin-lattice relaxation rate 1/ T 1 for various x of BaFe 2− x Ni x As 2 . The solid and dashed arrows indicate T c and T N , respectively. The error bar is the s.d. in fitting the nuclear magnetization recovery curve. Full size image Next, we use 75 As NMR to study the structural phase transition. A tetragonal-to-orthorhombic structural transition was found in the parent compound [25] , but no direct evidence for such structural transition was obtained in the doped BaFe 2− x Ni x As 2 thus far. In BaFe 2− x Co x As 2 , a structural transition was detected in the low-doping region [26] , but it is unclear how the transition temperature T s would evolve as doping level increases. The 75 As nucleus has a nuclear quadrupole moment that couples to the electric field-gradient (EFG) V xx (α= x , y , z ). Therefore, the 75 As-NMR spectrum is sensitive to a structural phase transition, as below T s the EFG will change appreciably. Such change was indeed confirmed in the parent compounds BaFe 2 As 2 (ref. 17 ) and LaFeAsO (ref. 27 ). When a magnetic field H 0 is applied in the ab plane, the NMR resonance frequency f is expressed by where m =3/2, 1/2 and −1/2, φ is the angle between H 0 and the a axis, ν Q is the nuclear quadrupole resonance frequency, which is proportional to the EFG, and . For a tetragonal crystal structure, η =0. For an orthorhombic structure, however, the a axis and b axis are not identical, which results in an asymmetric EFG so that η >0. Therefore, for a twined single crystal, the field configurations of H 0 || a axis ( φ =0°) and H 0 || b axis ( φ =90°) will give a different f m ↔ m −1 ( φ , η ), leading to a splitting of a pair of the satellite peaks into two. The above argument also applies to the case of electronic nematic phase transition such as orbital ordering, as the EFG is also sensitive to a change in the occupation of the on-site electronic orbits. As shown in Fig. 7a,b , only one pair of satellite peaks is observed at high temperature for both x =0.05 and 0.07. Below certain temperature, T s , however, we observed a splitting of the satellite peaks. This is strong microscopic evidence for a structural transition occurring in the underdoped samples, where the NMR spectra split owing to the formation of the twinned orthorhombic domains. In fact, each satellite peak can be well reproduced by assuming two split peaks. The obtained T s =90 K for x =0.05 and T s =70 K for x =0.07 agrees well with the resistivity data where an upturn at T s is observed, see Fig. 8 . This feature in the spectra persists to the higher dopings x =0.10 and 0.12. For the optimal doping x =0.10, the spectrum is nearly unchanged for 40 K≤ T ≤60 K, but suddenly changes at 20 K. This indicates that a structural transition takes place below T s =~40 K for this doping composition. For x =0.12, the two satellite peaks do not change at high temperatures, but shift to the opposite direction below T =10 K. Each broadened peak at T =6 K can be well fitted by a superposition of two peaks. This is the first observation that a structural phase transition takes place below T c . For x =0.14, however, no broadening of the spectra was found down to T =4.5 K; the spectrum shift to the same direction is due to a reduction of the Knight shift in the superconducting state. This indicates that T s =0 around x c2 =0.14. The T s results obtained by NMR are summarized in the phase diagram as shown in Fig. 2b . 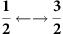Figure 7: The satellite peaks corresponding to theandtransitions. (a–d) The satellite peaks with the external fieldH0applied along theaaxis orbaxis above and belowTsforx=0.05, 0.07, 0.10 and 0.12. The peaks split belowTsdue to a change in EFG. All the spectra are fitted by a single Gaussian function aboveTs, but by two Gaussian functions belowTs. (e) The satellite peaks forx=0.14, which only shift to the same direction due to a reduction of the Knight shift as inFig. 3c. Figure 7: The satellite peaks corresponding to the and transitions. ( a – d ) The satellite peaks with the external field H 0 applied along the a axis or b axis above and below T s for x =0.05, 0.07, 0.10 and 0.12. The peaks split below T s due to a change in EFG. All the spectra are fitted by a single Gaussian function above T s , but by two Gaussian functions below T s . ( e ) The satellite peaks for x =0.14, which only shift to the same direction due to a reduction of the Knight shift as in Fig. 3c . 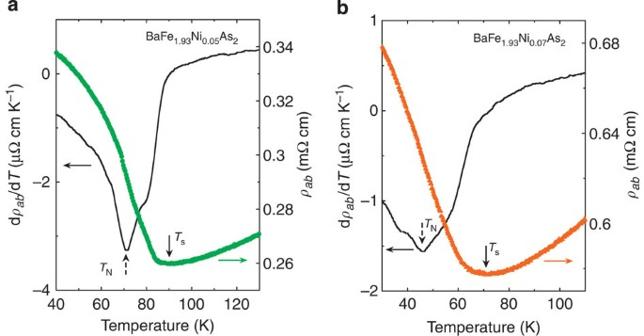Figure 8: The enlarged part of the electrical resistivity and its derivative for the underdoped samples. (a) Enlarged part of the in-plane electrical resistivityρab(right vertical axis) and its derivative (left vertical axis) forx=0.05. (b) Data forx=0.07. The solid and dashed arrows indicate the structural phase transition temperatureTsand the antiferromagnetic transition temperatureTNdetermined by NMR, respectively. Full size image Figure 8: The enlarged part of the electrical resistivity and its derivative for the underdoped samples. ( a ) Enlarged part of the in-plane electrical resistivity ρ ab (right vertical axis) and its derivative (left vertical axis) for x =0.05. ( b ) Data for x =0.07. The solid and dashed arrows indicate the structural phase transition temperature T s and the antiferromagnetic transition temperature T N determined by NMR, respectively. Full size image Therefore, the minimal n =1.1 of the resistivity exponent around x c2 implies quantum critical fluctuations associated with the structural QCP. We hope that our work will stimulate more experimental measurements such as elastic constant, which is also sensitive to such critical fluctuations [28] . It should be emphasized here that the exponent n =1.1 is smaller than n =4/3 expected for the fluctuations dominated by q =(0,0) (ref. 12 ). Our result suggests that the fluctuation associated with x c2 is local (namely, all wave vectors contribute to the quasiparticles scattering), which would lead to an n =1 (ref. 29 ). The mechanism for the superconductivity in iron-pnictides has been discussed in relation to magnetic fluctuations [30] , [31] , [32] as well as structural/orbital fluctuations [33] . In this context, it is worthwhile noting that T c is the highest around x c1 . This suggests that the superconductivity in BaFe 2− x Ni x As 2 is more closely related to the antiferromagnetic QCP rather than the structural QCP. Also, previous results suggestive of a magnetic QCP was reported for BaFe 2 (As 1− x P x ) 2 (refs 34 , 35 ), but isovalent P substitution for As does not add carriers there. In the present case, Ni directly donates electrons into the system (chemical doping), so the tuning parameter is totally different here. Thus, our work demonstrates that BaFe 2− x Ni x As 2 is a new material that provides a unique opportunity to study the issues of quantum criticality. In particular, our result suggests that x c2 is a new type of QCP at which the exponent n cannot be explained by existing theories. Although the importance of the tetragonal-to-orthorhombic structural transition, which is often associated with electronic nematicity [36] , [37] , has been pointed out in the pnictides [33] , [38] , [39] , the physics of a QCP associated with it is a much less-explored frontier, which deserves more investigations in the future. Sample preparation and characterization The single crystal samples of BaFe 2− x Ni x As 2 used for the measurements were grown by the self-flux method [40] . Here the Ni content x was determined by energy-dispersive x-ray spectroscopy. The T c was determined by DC susceptibility measured by a superconducting quantum interference device with the applied field 50 Oe parallel to the ab plane. The T c is 3.5, 14, 18.5, 18.2, 16.8 and 13.1 K for x =0.05, 0.07, 0.09, 0.10, 0.12 and 0.14, respectively. The resistivity measurements Resistivity measurements were performed in quantum design physical properties measurement system by a standard dc four-probe method. Here we have used the same single crystals used in the NMR measurements. The electrical resistance was measured upon both warming and cooling processes in order to ensure no temperature effect from the electrodes on the samples. Both the warming and the cooling speed is 2 K min −1 . Measurements of NMR spectra and T 1 The NMR spectra were obtained by integrating the spin echo as a function of the RF frequency at a constant external magnetic field H 0 =11.998 T. The nucleus 75 As has a nuclear spin I =3/2 and the nuclear spin Hamiltonian can be expressed as where γ /2 π =7.9219 MHz T −1 is the gyromagnetic ratio of 75 As, h is Planck constant, H int is the internal magnetic field at the As nuclear spin site resulting from the hyperfine coupling to the neighbouring Fe electrons. The T 1 was determined by using the saturation-recovery method and the nuclear magnetization is fitted to , where M ( t ) is the nuclear magnetization at time t after the saturation pulse [41] . The curve is fitted very well and T 1 is of single component. Simulation of the spectra In order to reproduce the spectra, we assume that the distribution of the internal magnetic field is Gaussian as, where I ( f ) is the intensity of the spectra, H σ is the distribution of the internal magnetic field H int , and ν c is the nuclear quadrupole resonance frequency tensor along the c axis. Then the spectrum is fitted by convoluting equation 3 with a Gaussian broadening function that already exists above T N . For n =0 (central transition), A 0 =1 and is the full-width at half maximum (FWHM) of the central peak above T N . For n =±1 (satellites), A ±1 =3/4 and is the FWHM of satellite lines above T N . The red solid curve in Fig. 3a is a fit with H σ =0.37 T, =0.03 MHz and =0.38 MHz, which was taken from the spectrum at T =100 K. The red solid curve in Fig. 3b is a fit with =0.04 MHz and =0.5 MHz, which was taken from the spectrum at T =50 K. How to cite this article: Zhou, R. et al . Quantum criticality in electron-doped BaFe 2− x Ni x As 2 . Nat. Commun. 4:2265 doi: 10.1038/ncomms3265 (2013).